Extreme sensitivity of graphene photoconductivity to environmental gases Graphene is a single layer of covalently bonded carbon atoms, which was discovered only 8 years ago and yet has already attracted intense research and commercial interest. Initial research focused on its remarkable electronic properties, such as the observation of massless Dirac fermions and the half-integer quantum Hall effect. Now graphene is finding application in touch-screen displays, as channels in high-frequency transistors and in graphene-based integrated circuits. The potential for using the unique properties of graphene in terahertz-frequency electronics is particularly exciting; however, initial experiments probing the terahertz-frequency response of graphene are only just emerging. Here we show that the photoconductivity of graphene at terahertz frequencies is dramatically altered by the adsorption of atmospheric gases, such as nitrogen and oxygen. Furthermore, we observe the signature of terahertz stimulated emission from gas-adsorbed graphene. Our findings highlight the importance of environmental conditions on the design and fabrication of high-speed, graphene-based devices. The experimental realization of graphene, a single layer of graphite, in 2004 (ref. 1 ) rapidly led to the observation of massless Dirac fermions and the half-integer quantum Hall effect [2] . Since then, many potential applications have been suggested [3] , [4] , and recently graphene-based touch-screen displays [5] , transistors [6] , [7] and integrated circuits [8] have been demonstrated. The high mobility of charge carriers in graphene makes it an ideal material for extremely high-speed devices [6] , [7] , indeed terahertz-frequency switching has been predicted [3] . The potential for the realization of such devices was greatly enhanced by the emergence of large-area graphene sheets grown by chemical vapour deposition (CVD) [9] . However, the design and production of these high-frequency devices require a fuller understanding of both non-equilibrium carrier dynamics in graphene [10] and its susceptibility to environmental conditions [11] . Ultrafast spectroscopic techniques provide an excellent probe of non-equilibrium carrier dynamics in graphene [12] . Ultrafast cooling and relaxation of photoexcited charge carriers in graphene have been observed using optical pump–optical probe spectroscopy. Several studies [10] , [13] , [14] have shown that graphene becomes more transparent at optical frequencies after intense photoexcitation (photo-induced bleaching), owing to state blocking of interband absorption. Furthermore, these studies showed that thermalization of photoexcited carriers occurs within tens of femtoseconds, and a subsequent cooling by carrier–phonon interactions occurs on a picosecond time scale. Although optical photons probe interband charge dynamics, terahertz frequency photons are excellent probes of intraband dynamics. Studies of intraband relaxation in graphene have been performed using optical pump–terahertz probe spectroscopy [12] , [15] , [16] , [17] . George et al. [15] revealed that the absorption of the terahertz photons in epitaxially grown graphene increases after intense (interband) optical excitation. The increase in absorption was attributed to an increase in the density of mobile charge carriers after photoexcitation. However, a comparable study on CVD-grown graphene found the opposite effect photo-induced bleaching [18] . It is known that CVD-grown graphene is p-doped, due to residual impurities and defects from the production process [19] , unlike epitaxial graphene [17] . Despite this, equilibrium carrier dynamics in CVD-grown graphene have been shown to be similar to other forms of graphene in the terahertz regime, suggesting that growth conditions cannot explain the discrepancy between the epitaxial and CVD graphene in the pump–probe studies [20] . In this study, we utilized terahertz time-domain spectroscopy to measure the photoconductivty of CVD-grown graphene in four different environment types: air, oxygen, nitrogen and vacuum. We demonstrate that CVD-grown graphene can display either photo-induced bleaching or photo-induced absorption, depending on the type and density of gas adsorbed on its surface. Our results highlight the dramatic effects environmental conditions have on the high-frequency electrical properties of graphene. These results have important implications for the design of future graphene electronic devices. In particular, the order-of-magnitude changes in photoconductivity we observe could provide a basis for precise graphene-based gas monitors. Conversely, the sensitivity of the opto-electronic properties of graphene to environmental conditions will need to be addressed during the design and fabrication of future devices. Sample preparation and characterization The CVD samples used in this study were grown on copper foil and transferred to z-cut quartz substrates using PMMA (poly(methyl methacrylate)) as a supporting layer (for details see the Methods section). Raman microscopy and atomic force microscopy (AFM) revealed that the samples were primarily a graphene monolayer with relatively few defects. A typical Raman spectrum is shown in Fig. 1 and exhibits a Lorentzian 2D Raman peak (2,700 cm −1 ), with the ratio of intensities of the 2D and G (1,580 cm −1 ) peaks, I 2D / I G ~2, which is indicative of monolayer growth. In addition, the relative weakness of the D peak (1,350 cm −1 ) demonstrates the small number of defects and low disorder in the samples, confirming their high quality [21] . Ultraviolet-visible absorption measurements revealed an absorption of ~πα, where α is the fine structure constant, also suggesting monolayer growth (see Supplementary Methods ) [22] . The AFM images ( Fig. 1b ) showed the graphene sheet thickness measured from the edge to be ~0.72 nm, further suggesting monolayer growth [23] . Hall measurements revealed the sample to be p-doped, with a hole density 8 × 10 12 cm −2 and Fermi level ε F ~−0.3 eV. 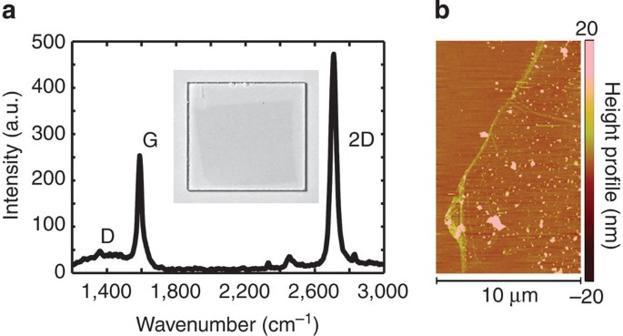Figure 1: Characterization of graphene samples. (a) Raman spectroscopy. The relative intensities of the 2D and G peaks suggest monolayer graphene21. Inset: photograph of graphene sheet with an area of 1 × 1 cm2on quartz. (b) Surface topography of CVD-grown graphene measured by AFM. The residuals remaining on graphene surface can be attributed to incomplete decomposition or carbonization of PMMA. Figure 1: Characterization of graphene samples. ( a ) Raman spectroscopy. The relative intensities of the 2D and G peaks suggest monolayer graphene [21] . Inset: photograph of graphene sheet with an area of 1 × 1 cm 2 on quartz. ( b ) Surface topography of CVD-grown graphene measured by AFM. The residuals remaining on graphene surface can be attributed to incomplete decomposition or carbonization of PMMA. Full size image Terahertz time-domain spectroscopy To assess the influence of atmospheric gas adsorption on graphene, we used terahertz spectroscopy. This technique allowed us to observe intraband charge dynamics and investigate the high-frequency electrical properties of graphene. Terahertz spectroscopy is ideal for electrically characterizing surface-sensitive materials such as graphene, as it is a non-contact technique and covers an important frequency range (~100 GHz to >3 THz) for high-speed device operation [24] . Optical pump–terahertz probe spectroscopy measurements were performed with CVD-grown graphene samples in an atmosphere of air, N 2 or O 2 , or in a vacuum. Before each set of measurements, the sample was left under a vacuum of 10 −5 mbar for 2 h to remove existing adsorbants (see Supplementary Methods for Langmuir coverage calculations). For the vacuum measurements, the graphene was left for a further 2 h with 800 nm (1.55 eV) ‘pump’ photons incident upon the sample before measurement. For the gaseous measurements, 1 bar of air, N 2 or O 2 , was introduced after 2 h under vacuum, and measurements were taken after a further 2 h, again with the ‘pump’ beam incident upon the sample. Measurements were found to be reproducible on different samples and were independent of sample history. That is, the effect of exposure to any of the gases could be ‘reset’ by placing the sample in vacuum for 2 h. For the measurements, the electric field of a terahertz pulse transmitted through the graphene was sampled after photoexcitation by an 800 nm, 180 μJ cm −2 fluence pump pulse, , and without the photoexcitation, . The photo-induced change in terahertz transmission of the sample, was recorded using lock-in detection. The principle of the measurements is illustrated in Fig. 2a . The terahertz pulse probes the photoexcited graphene sample at a time t 2 after photoexcitation. The terahertz probe is then mapped out in time by varying the difference in time of arrival, t 1 , between the terahertz pulse and an 800-nm gate pulse at an electro-optic detection crystal (GaP). 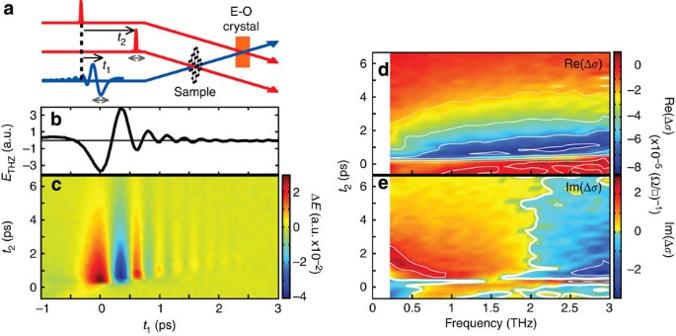Figure 2: Terahertz spectroscopy of graphene in O2. (a) Schematic representation of the measurement. Varyingt1allows the electric field,ETHz, of the terahertz probe pulse to be sampled in the electro-optic (E-O) crystal. The sample can be probed at different times after photoexcitation by alteringt2. (b,c) Terahertz electric field,ETHz, transmitted through the sample (b), and the corresponding photo-induced change in transmission, ΔE(c), as a function of the pump–probe delay time,t2. (d,e) Real (d) and imaginary (e) parts of the frequency-dependent photoconductivity as a function oft2. The contours highlight increments of 2 × 10−5(Ω/)−1. The thicker contour in e represents Im(Δσ)=0, corresponding to the Lorentzian peak frequency,ω0. Measurements were performed in pure oxygen at room temperature and pressure. Figure 2: Terahertz spectroscopy of graphene in O 2 . ( a ) Schematic representation of the measurement. Varying t 1 allows the electric field, E THz , of the terahertz probe pulse to be sampled in the electro-optic (E-O) crystal. The sample can be probed at different times after photoexcitation by altering t 2 . ( b , c ) Terahertz electric field, E THz , transmitted through the sample ( b ), and the corresponding photo-induced change in transmission, Δ E ( c ), as a function of the pump–probe delay time, t 2 . ( d , e ) Real ( d ) and imaginary ( e ) parts of the frequency-dependent photoconductivity as a function of t 2 . The contours highlight increments of 2 × 10 −5 (Ω/ ) −1 . The thicker contour in e represents Im(Δ σ )=0, corresponding to the Lorentzian peak frequency, ω 0 . Measurements were performed in pure oxygen at room temperature and pressure. Full size image In Fig. 2b we present the measured terahertz electric field, E THz , transmitted through graphene in a pure oxygen atmosphere and the corresponding change in transmission due to photoexcitation, Δ E . The induced Δ E decreases as the delay between pump and probe, t 2 , is increased. The photo-induced change in terahertz transmission is seen to decay within ~5 ps. Further information may be extracted from these data by performing a Fourier transform on the electric field data to give directly the frequency-dependent complex photoconductivity, Δ σ ( ω ), without resorting to the Kramers–Kronig relations, via [17] where Z 0 is the impedance of free space, Z 0 =377 Ω and n s is the refractive index of the quartz substrate, n r =2.1 ( [25] ) at terahertz frequencies. Figure 2d show the real and imaginary parts of the photoconductivity, respectively, as a function of the pump–probe delay time. To more easily compare the photoconductivity in different atmospheres, we take slices of the data from Fig. 2 and the corresponding data for the other environment types. For instance, holding t 1 constant at the maximum terahertz electric field (for example, t 1 =0 in Fig. 2c ) and observing the resulting Δ E as pump–probe delay time t 2 is varied yields an optical pump–terahertz probe measurement, which provides the average terahertz response of the sample. In Fig. 3 , we plot −Δ E / E THz , which is proportional to the photoconductivity of the graphene, as a function of the delay time between the pump and probe pulses in the four atmosphere types. It should be noted that because of the large number of holes already present near the Dirac point in this p-doped sample, the transient response probed by the terahertz is dominated by electron dynamics. 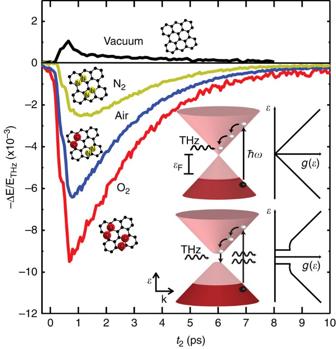Figure 3: Environmental dependence of pump-induced change in terahertz photoconductivity. Here,. From top to bottom: graphene in vacuum, N2, air and O2at room temperature. Photo-induced absorption is observed in vacuum, but photo-induced bleaching is observed in gaseous environments. Inset: schematic representation of the pump–probe measurements of p-doped graphene (εF~0.3 eV) in vacuum (top) and in the presence of gases (bottom), with corresponding density of states (g(ε)). The high-energy pump () excites carriers far above the Dirac point, which cool by phonon emission. In gapless graphene, terahertz photons can be absorbed by the photoexcited carriers. In the presence of gases, stimulated emission releases extra terahertz photons, yielding a bleaching pump–probe signal. Figure 3: Environmental dependence of pump-induced change in terahertz photoconductivity. Here, . From top to bottom: graphene in vacuum, N 2 , air and O 2 at room temperature. Photo-induced absorption is observed in vacuum, but photo-induced bleaching is observed in gaseous environments. Inset: schematic representation of the pump–probe measurements of p-doped graphene ( ε F ~0.3 eV) in vacuum (top) and in the presence of gases (bottom), with corresponding density of states ( g (ε)). The high-energy pump ( ) excites carriers far above the Dirac point, which cool by phonon emission. In gapless graphene, terahertz photons can be absorbed by the photoexcited carriers. In the presence of gases, stimulated emission releases extra terahertz photons, yielding a bleaching pump–probe signal. Full size image Immediately after photoexcitation in vacuum, the terahertz conductivity increases (photo-induced absorption) within 1 ps, and subsequently relaxes with two distinct time scales. Initially, fast cooling occurs within ~0.6 ps and a longer, exponential cooling occurs with a time scale of ~2.5 ps. Such a relaxation is consistent with other studies, which associated the first rapid cooling with emission of optical phonons, followed by a bottleneck when the carrier temperature cools below the hot optical phonon temperature (~0.196 and 0.162 eV (ref. 16 )), slowing further cooling [10] , [14] , [16] . However, when graphene is placed in a gaseous atmosphere, the photo-induced change is dramatically different. Surprisingly, the photoconductivity signal flips from being purely positive in vacuum to purely negative in all the gas environments. Following photoexcitation in air, N 2 or O 2 , the terahertz conductivity decreases within 1 ps, and then relaxes with a common monoexponential time scale of 2.5 ps. The similarity between this time constant and that of cooling in vacuum suggests the continued importance of the carrier–phonon interactions. Adsorbed O 2 was found to have the strongest influence on charge dynamics in graphene, with the negative photoconductivity almost an order of magnitude greater than the induced absorption under vacuum. A negative transient absorption, such as we observe, may be attributed to either stimulated emission in the samples or a bleaching effect. To understand more about the origin of the negative photoconductivity, it is informative to consider the photoconductivity spectra at a fixed time after photoexcitation. 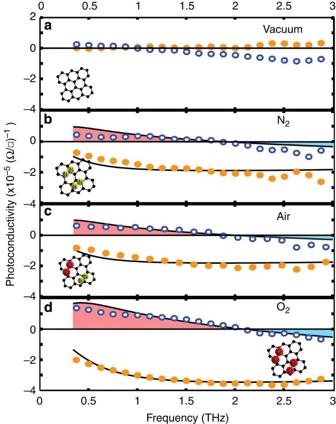Figure 4: Photoconductivity spectra of graphene in different environments. (a–d) Photoconductivity in vacuum (a), N2(b), air (c) and O2(d), taken at 2 ps after photoexcitation by the optical pump. Solid orange dots show the real part of the photoconductivity, hollow blue dots show the imaginary part. The solid black line inb–dis a Lorentzian model fit to the conductivity data, demonstrating the Lorentzian form the of photoconductivity in gaseous environments. Shading is used to emphasize the change from positive to negative Im(Δσ). This point corresponds to the peak Lorentzian frequency,ω0. Figure 4 shows the photoconductivity in all four atmosphere types at 2 ps after photoexcitation ( t 2 =2 ps). The spectrum of graphene in vacuum reveals a relatively flat and positive real part of photoconductivity, in stark contrast to the strongly negative (real) photoconductivity seen for gas-absorbed graphene. Furthermore, the spectral photoconductivity of graphene samples in the presence of N 2 , air and O 2 can be seen to exhibit a Lorentzian form, Figure 4: Photoconductivity spectra of graphene in different environments. ( a – d ) Photoconductivity in vacuum ( a ), N 2 ( b ), air ( c ) and O 2 ( d ), taken at 2 ps after photoexcitation by the optical pump. Solid orange dots show the real part of the photoconductivity, hollow blue dots show the imaginary part. The solid black line in b – d is a Lorentzian model fit to the conductivity data, demonstrating the Lorentzian form the of photoconductivity in gaseous environments. Shading is used to emphasize the change from positive to negative Im(Δ σ ). This point corresponds to the peak Lorentzian frequency, ω 0 . Full size image where Γ is the linewidth and ω 0 is the resonant frequency. The solid lines in Fig. 4 represent a least square fit of equation 2 to the experimental data. The fitted resonant frequency for graphene in air and N 2 was found to be ω 0 ~1.8 THz compared with ω 0 ~2 THz for graphene in an O 2 environment. The resonance in all gas types is spectrally very broad; the fitted linewidth was Γ~10 THz, independent of the gas type. The Lorentzian fit begins to deviate from the measured photoconductivity at low frequencies. The deviation is most noticeable for O 2 -exposed graphene ( Fig. 4d ). The non-zero value of Re(Δ σ ) evident in the data at low frequency suggests an underlying Drude-like response; however, inclusion of a Drude term does not enhance the fit within our observable bandwidth, and so has been neglected. In contrast, the photo-induced absorption in vacuum leads to a small, positive, spectrally flat, real conductivity, with a non-negligible imaginary part. A negative transient absorption signal with a Lorentzian lineshape is characteristic of stimulated emission. Hence, our data provide evidence that stimulated emission of terahertz photons is occurring in photoexcited graphene in the presence of atmospheric gases. Theoretical studies have predicted amplified stimulated emission of terahertz radiation from sufficiently intensely photoexcited graphene [26] . The proposed mechanism is that after photoexcitation, the charge carriers relax and populate states around the Dirac point from where they can radiatively recombine. Thus, terahertz emission over a large spectral range is expected to be possible [26] . Although our measurements do not show amplification of the terahertz probe (losses are still greater than gain), stimulated terahertz emission below the gain threshold is consistent with our observations. We now consider the mechanism for the dramatic changes of photoconductivity in graphene under different gas environments. The ability to ‘reset’ the effects of gas exposure by placing the graphene samples in vacuum for 2 h (at room temperature) suggests that the gas molecules are physisorbed rather than chemisorbed to the graphene surface. Physisorption of O 2 and N 2 on graphene could act as a dopant [27] , lead to the opening of a small band gap at the Dirac point [28] , [29] and/or lead to a modification of the density of states [30] , [31] . Hall measurements (see Methods) showed only 3% changes in the Fermi level after gas adsorption, indicating that doping alone is unlikely to account for the huge change in photoconductivity we observe. The opening of an ~8-meV band gap on gas adsorption and associated increase in the density of electron and hole states near the band extrema would be consistent with our observations. In this case, electrons injected into the conduction band by 800 nm (1.55 eV) photoexcitation would relax rapidly to near the band minimum via phonon-mediated processes, as shown on the inset of Fig. 3 . Recombination for the photoinjected electrons across the band gap with a sea of holes would lead to the observed stimulated emission signal. The spectral broadness (Γ~10 THz) of the observed transition may then be explained by a combination of the following factors: a high interband transition rate (lifetime broadening), fast dephasing via electron–electron interactions and a cooling bottleneck below the optical phonon energies. However, full ab-inito calculations would be required to confirm the exact mechanism. Note that as the CVD graphene is heavily p-doped, the opening of a band gap is not directly observable by terahertz transmission spectroscopy, as there are no electrons near the band gap to be excited by the low-energy terahertz photons (see Supplementary Discussion and inset of Fig. 3 ). The adsorption of molecules on graphene would locally open a band gap and hence alter the otherwise linear density of states ( g (ε)) of the graphene, thereby increasing g (ε) at the top of the valance band and bottom of the conduction band (see inset of Fig. 3 ) [31] . However, a gap would only be opened in regions around adsorbed gas molecules, creating islands of semiconducting graphene amongst the unaltered, gapless graphene (see Supplementary Methods for Langmuir coverage calculations). As the terahertz probe is much larger than these puddles, the observed photoconductivity behaviour is the result of an interaction with both types of graphene. Increased stimulated emission will therefore be observed if gas molecules are more effectively adsorbed on the surface, thus creating a higher proportion of semiconducting material. Of the gases used in this study, O 2 is most likely to interact with graphene [32] , [33] , which is consistent with the increased negative photoconductivity signal observed in pure O 2 compared with air and N 2 . There are a number of other possible explanations for a Lorentzian photoconductivity in graphene. A positive Lorentzian conductivity may originate from the excitation of plasmons [34] . Terahertz surface plasmons have been predicted theoretically [35] , [36] and recently observed in spatially confined graphene [37] . However, the peak frequency of a plasmon-dependent conductivity varies with carrier concentration as ω 0 n 1/4 (ref. 37 ), and Re(Δ σ ) is expected to be positive in contrast to our experiments. Figure 2 demonstrates that our measured ω 0 does not decrease with time after photoexcitation, and hence is independent of photoexcited carrier concentration. Additional measurements showed ω 0 to be independent of pump fluence (see Supplementary Discussion ). Thus, it is unlikely that excitation of plasmons explains the Lorentzian response. A negative photoconductivity may also be attributed to a photo-induced reduction in conductivity, for example, by an increase in the carrier–carrier or carrier–phonon (intraband) scattering rates. However, it is not clear why such mechanisms would produce a Lorentzian form or occur only in gas-adsorbed graphene. Finally, ground-state bleaching could lead to a negative photoconductivity with Lorentzian form; however, the states associated with the absorption of (1.55 eV) optical photons in graphene are well separated from the states near the Dirac point that are associated with interband terahertz absorption and emission (see the inset of Fig. 3 ). We therefore conclude that the opening of a small band gap in the presence of adsorbed gas molecules is the most likely explanation for our measurements. In summary, we have used terahertz time-domain spectroscopy to non-invasively probe photoexcited carrier dynamics in CVD-grown graphene. We have observed that gas adsorption can dramatically alter the high-frequency electrical response of graphene sheets. We also provide experimental evidence for stimulated emission of terahertz photons in graphene. Furthermore, our results demonstrate the huge influence environmental factors can exert on the behaviour of hot carriers in CVD graphene, and highlight the importance of consideration of such factors for future CVD graphene opto-electronic devices. Synthesis and transfer of CVD graphene Large-area graphene films were prepared by CVD on 25 μm copper foil (Alfa Aesar). Before the growth, the copper foil was heated in hydrogen from room temperature to 1,000 °C for 60 min for removal of surface oxides. As temperature reached 1,000 °C, a mixed flow of H 2 (15 sccm) and CH 4 (60 sccm) was introduced for graphene growth. After CVD, the graphene film was separated from copper foil and then attached to the z-cut quartz substrate by the polymer transfer process: PMMA; MicroChem Co., NANO PMMA 950K A4) was spin-coated on graphene/copper foil to form a protective layer. The copper foil was etched at 25 °C in ferric nitride solution (50 g l −1 , J.T. Baker ACS reagent, 98%), leaving a transparent PMMA/graphene film floating on the solution. After rinsing, the film was transferred onto the quartz substrate and the PMMA capping layer was dissolved in acetone at 60 °C overnight. To remove the residual PMMA, graphene films were annealed at 450 °C at 500 Torr in the mixed gases of H 2 (20 sccm) and Ar (80 sccm) for decomposition of the polymer. Characterization Primary characterization of the sample was performed by Raman spectroscopy [21] , using an NT-MDT confocal Raman microscopic system (laser wavelength 473 nm, power 0.5–1 mW, spot size 0.5 μm). Additional characterization was performed using ultraviolet-visible absorption spectroscopy (Perkin-Elmer Lambda 9 UV-visible-NIR Spectrophotometer) in the range 500–1,300 nm, confirming the expected constant πα absorption of a single layer of graphene in this wavelength range [22] . Nominally identical samples were characterized using AFM (Veeco Dimension-Icon) and room temperature Hall effect measurements based on the van der Pauw method (3S Co., NI PXI-1033). From the Hall effect measurements averaged across eight samples, the sheet resistance, carrier density and Hall mobility were found to be 1,100±350 Ω/□, 8±2 × 10 12 cm −2 and 800±250 cm 2 V s −1 , respectively. The characterizations show that the quality of the graphene samples is fairly good. Further Hall effect measurements were performed to examine the equilibrium electrical properties of the graphene samples under different gaseous environments. Two systems were used for the measurements, one based on a permanent magnet (0.68 T), and another using a swept electromagnet (0–0.91 T). Samples were held in a vacuum vessel, which could be purged with different gasses. The Fermi levels were deduced using the relation , where v F ≈10 6 ms −1 (ref. 2 , 37 ). The equilibrium carrier density, and hence Fermi level, were found to be relatively insensitive to the gaseous environment, with variations in n and ε F between samples being greater than changes induced by the gases. It was found that compared with vacuum conditions, exposure to pure nitrogen gas decreased the carrier density by ~5%, exposure to oxygen increased the carrier density by ~7% and exposure to air increased it by ~3%, correspnding to Fermi level changes of ~2%, ~3% and ~1%, respectively. These changes are consistent with previous observation of oxygen and nitrogen exposure doping CVD graphene p-type and n-type, respectively [27] , [38] . Terahertz spectroscopy A Ti:sapphire regenerative amplifier (Spectra-Physics Spitfire Pro) was used as the pulse laser source for both terahertz generation and optical pumping of the sample: 800 nm, 45 fs pulse duration, 5 kHz repetition rate and 4 W average power. Of this beam, 2.9 W, reduced to 0.29 W with a neutral density filter, was used to photoexcite the graphene sample, with a maximum fluence of 180 μJ cm −2 incident upon the sample, and beam width 2 mm. A fraction (200 μJ per pulse) of the amplifier beam was used to generate the terahertz probe beam by optical rectification [24] in a 2-mm GaP crystal. The terahertz beam had a width of 0.48 mm at the sample position. The area of graphene probed by the terahertz beam was much smaller than the area photoexcited by the pump beam; thus, the probe measured an area of roughly constant photoexcited carrier density. The remainder of the amplifier beam (16 μJ per pulse) was used as a gate beam for electro-optic sampling [24] of the terahertz field in a 200-μm GaP crystal. The terahertz electric field, E THz , was detected by a balanced photodiode circuit, and the signal extracted using a lock-in amplifier (Stanford Research SR830), referenced to a 2.5-kHz chopper in the terahertz generation beam. A further lock-in (SR830) was used to detect the optical pump-induced change in E THz , Δ E , by referencing to a 125-Hz chopper in the sample pump beam. The gaseous atmospheres used in the terahertz measurements were ambient air, 99.998% pure oxygen-free N 2 and 99.99% pure O 2 . A vacuum of 10 −5 mbar, generated using an oil-free pumping system (turbo molecular pump and scroll pump), was used for both the vacuum measurements and to remove adsorbants from the sample before gaseous measurements. How to cite this article: Docherty, C. J. et al. Extreme sensitivity of graphene photoconductivity to environmental gases. Nat. Commun. 3:1228 doi: 10.1038/ncomms2235 (2012).